Momentum-resolved hidden-order gap reveals symmetry breaking and origin of entropy loss in URu2Si2 Spontaneous symmetry breaking in physical systems leads to salient phenomena at all scales, from the Higgs mechanism and the emergence of the mass of the elementary particles, to superconductivity and magnetism in solids. The hidden-order state arising below 17.5 K in URu 2 Si 2 is a puzzling example of one of such phase transitions: its associated broken symmetry and gap structure have remained longstanding riddles. Here we directly image how, across the hidden-order transition, the electronic structure of URu 2 Si 2 abruptly reconstructs. We observe an energy gap of 7 meV opening over 70% of a large diamond-like heavy-fermion Fermi surface, resulting in the formation of four small Fermi petals, and a change in the electronic periodicity from body-centred tetragonal to simple tetragonal. Our results explain the large entropy loss in the hidden-order phase, and the similarity between this phase and the high-pressure antiferromagnetic phase found in quantum-oscillation experiments. The heavy-fermion material URu 2 Si 2 undergoes a second-order phase transition at T HO =17.5 K to a so-called hidden-order (HO) state whose order parameter is still unknown after almost 30 years of continued research [1] , [2] , [3] , [4] , [5] , [6] , [7] , [8] , [9] , [10] , [11] , [12] , [13] , [14] , [15] , [16] , [17] , [18] , [19] , [20] , [21] , [22] , [23] , [24] . Macroscopically, this transition is characterized by a large entropy loss and an energy gap of ~10 meV in the density of states at the Fermi level [3] , [5] , [6] , [23] . Microscopically, the paramagnetic (PM) state above T HO in URu 2 Si 2 is characterized by the existence of weak quasi-elastic spin fluctuations at the commensurate wave vector Q 0 =(1,0,0) (reciprocal lattice units in the simple-tetragonal zone) and strong damped magnetic excitations at the incommensurate wave vector Q 1 =(1±0.4,0,0). The HO transition is accompanied by the development of an energy gap of ~4.5 meV in the spin excitations at Q 1 and the onset of a sharp inelastic signal (gap ~2 meV) of magnetic excitations at Q 0 [4] , [10] , [11] . From an electronic structure standpoint, angle-resolved photoemission spectroscopy (ARPES) experiments detected Fermi-surface pockets at the Γ, Z and X points of the Brillouin zone in the PM state [8] , [14] . In addition, high-resolution ARPES and scanning tunnelling microscopy experiments demonstrated that a Fermi-surface instability of itinerant heavy quasi-particles takes place at the transition [14] , [16] , [17] , [18] , [22] . However, a complete determination of the heavy-fermion Fermi-surface of URu 2 Si 2 , of its changes across the HO transition and a direct observation of the location and momentum dependence of the HO gap around the Fermi surface are still pressing unsolved questions. Here, by using high-resolution ultra-low-temperature ARPES over the three-dimensional (3D) reciprocal space of URu 2 Si 2 , we provide a direct experimental answer to these puzzles. 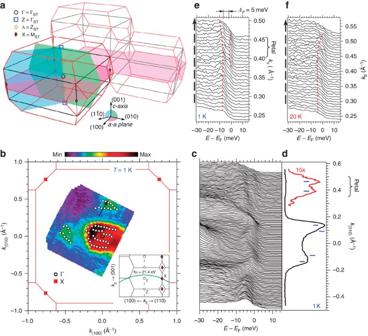Figure 1: Hidden-order Fermi petals and energy gapping along (100) (a) Body-centred tetragonal (BCT, red lines) and simple-tetragonal (ST, black lines) Brillouin zones for URu2Si2, showing their stacking in 3D reciprocal space, and some of the main high-symmetry points and directions. Henceforth, in this study the BCT Brillouin zone is represented by red (solid or dashed) lines and the ST Brillouin zone is represented by black lines. (b) Fermi surface map in thea−aplane of URu2Si2at 1 K. The open circles show the experimental Fermi momenta, determined from fits to momentum distribution curves (MDCs) atEF. (c) Raw energy distribution curves (EDCs) measured along the (010) direction through Γ inb. (d) Corresponding raw momentum distribution curve (MDC) atEF. The red curve is a 15-times magnification of the MDC at the petal. Vertical bars show the Fermi momenta of the inner square, outer square and petal. (e,f) Enlarged view of the raw EDCs around the petal, along the dashed black arrow inb), measured at 1 and 20 K, respectively. Dashed red lines are guides to the eye. At 1 K, the data show a gapΔP≈5 meV between a lower heavy band, originating from the central squares, and the upper electron pocket forming a Fermi petal. The gap closes at 20 K. All data in this figure were measured athν=21.4 eV. In 3Dk-space, this corresponds to the spherical surface represented by the green arc in the inset ofb. HO gap and related Fermi-surface reconstruction Figure 1a serves as a convenient guide to the 3D reciprocal space in URu 2 Si 2 , to help navigate through the data presented in this work. Measurements at fixed photon energy ( hν ) give the electronic structure along the a − a plane at fixed k ‹001› , whereas measurements as a function of photon energy provide the electronic structure in the a − c plane (see Methods). All throughout this paper, the low-temperature spectra were taken at 1 K. URu 2 Si 2 undergoes a superconducting transition at ~1.2 K (ref. 1 ), showing a superconducting gap of the order of 0.15 meV at 1 K (ref. 25 ), at least 30 times smaller than our resolution (Methods). Hence, any changes that might be induced by the superconducting transition do not affect our discussions. We indeed checked that apart from thermal broadening, the spectra at 1 and 5 K are identical (see Supplementary Fig. 1 and Supplementary Note 1 ). Figure 1: Hidden-order Fermi petals and energy gapping along (100) ( a ) Body-centred tetragonal (BCT, red lines) and simple-tetragonal (ST, black lines) Brillouin zones for URu 2 Si 2 , showing their stacking in 3D reciprocal space, and some of the main high-symmetry points and directions. Henceforth, in this study the BCT Brillouin zone is represented by red (solid or dashed) lines and the ST Brillouin zone is represented by black lines. ( b ) Fermi surface map in the a − a plane of URu 2 Si 2 at 1 K. The open circles show the experimental Fermi momenta, determined from fits to momentum distribution curves (MDCs) at E F . ( c ) Raw energy distribution curves (EDCs) measured along the (010) direction through Γ in b . ( d ) Corresponding raw momentum distribution curve (MDC) at E F . The red curve is a 15-times magnification of the MDC at the petal. Vertical bars show the Fermi momenta of the inner square, outer square and petal. ( e , f ) Enlarged view of the raw EDCs around the petal, along the dashed black arrow in b ), measured at 1 and 20 K, respectively. Dashed red lines are guides to the eye. At 1 K, the data show a gap Δ P ≈5 meV between a lower heavy band, originating from the central squares, and the upper electron pocket forming a Fermi petal. The gap closes at 20 K. All data in this figure were measured at hν =21.4 eV. In 3D k -space, this corresponds to the spherical surface represented by the green arc in the inset of b . Full size image Figure 1b presents the Fermi surface at 1 K in the a − a plane around Γ. The data show two central square-like Fermi-surface sheets surrounded by four smaller half-circles, henceforth called ‘Fermi petals’, along the (100) and equivalent directions. The central squares originate from an ‘M’-shaped heavy band, shown in the raw spectra of Fig. 1c , which is cut by the Fermi level slightly below the tips of the ‘M’, thus crossing E F twice [22] . The Fermi petals represent one of the crucial new discoveries of this work. As seen from Fig. 1c,d , they correspond to small electron pockets and present a gap of Δ P ≈5 meV with respect to the hole-like wings of the band forming the inner squares. The distance between the centre of two opposite petals is 0.91±0.01 Å −1 . It is worth noting that this corresponds, in reciprocal-lattice units, to the incommensurate excitation vector Q 1 =(0.6,0,0) observed in inelastic neutron scattering experiments [4] , [10] (see Methods). Thus, our data suggest a possible link, which should be investigated in future theoretical and experimental works, between the electronic structure around the petals and the incommensurate inelastic spin excitations at Q 1 . More important, as shown in Fig. 1e,f , in the PM state at 20 K the gap forming the Fermi petals is not observed anymore within our resolution. The heavy band there now crosses E F , giving rise, as we will see next, to a larger Fermi surface in the PM state. 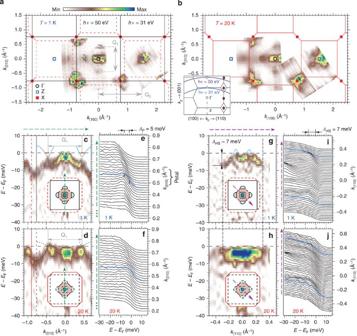Figure 2: Fermi-surface gapping and electronic reconstruction. (a,b) In-plane Fermi surface maps at 1 and 20 K spanning the Γ,ZandXpoints. Each map combines data measured at 31 and 50 eV, reaching different points in the Brillouin zone as shown in the inset ofb. The double arrows show the vectorsQ1, connecting two Fermi petals, andQ0, corresponding to a ST electronic periodicity. Open circles show the Fermi momenta from data inFig. 1. (b,c,d) ARPES dispersions (second derivative) at 1 and 20 K, respectively, measured along the (010) direction as shown by the dashed green arrows in the insets. The black and red lines denote, respectively, the borders of the ST and BCT Brillouin zones. Blue curves incand dashed brown curves indare guides to the eye. Incthe orange dashes mark the experimental location of the petals, whose intensity is too small to be apparent in this figure. (e,f) Raw energy distribution curves (EDCs) from (c,d) zooming into the region where the petals form. Spectra in blue correspond tok||=±|Q1|/2. (g,h) Same ascanddmeasured along (110) as shown by the dashed purple arrows in the insets. Dashed black lines are the Fermi momenta in the PM state. The blue curve ingis a fit serving as a guide to the eye22. (i,j) Raw EDCs fromgandh. Spectra in blue show the Fermi momenta in the PM state. Figure 2a,b present a complete view of the changes at the in-plane Fermi surface over the Γ, Z and X points— c.f. pink plane in Fig. 1a . At 1 K, in Fig. 2a , one sees the Fermi petals around Γ. The transition to the PM state, in Fig. 2b , comes with the formation of a large diamond-like Fermi surface of diagonals ~| Q 1 | along (100) and (010), instead of the petals present in the HO state. In fact, Fig. 2c–f show that the petals along (100) originate from the anti-crossing of two bands occurring at k ‹100› =±| Q 1 |/2. In the HO state, Fig. 2c,e , the anti-crossing gap is Δ P ≈5 meV, as already described in Fig. 1 . In the PM state, within our resolution, the above bands disperse through E F approximately at their crossing point (±| Q 1 |/2) and the gap forming the petals is not observed anymore: it has either closed or shifted above E F . Fig. 2g–j show that this dramatic reconstruction of the Fermi surface is accompanied by the closing, in the PM state, of a large gap Δ HS ≈7 meV around ‘hotspots’ of Fermi momenta k F ≈±0.3 Å −1 in the (110) direction. As seen in Fig. 2a , the ‘hotspots’ are actually ‘hot arcs’, gapping all the region between two petals in the ordered state. Figure 2: Fermi-surface gapping and electronic reconstruction. ( a , b ) In-plane Fermi surface maps at 1 and 20 K spanning the Γ, Z and X points. Each map combines data measured at 31 and 50 eV, reaching different points in the Brillouin zone as shown in the inset of b . The double arrows show the vectors Q 1 , connecting two Fermi petals, and Q 0 , corresponding to a ST electronic periodicity. Open circles show the Fermi momenta from data in Fig. 1 . ( b , c , d ) ARPES dispersions (second derivative) at 1 and 20 K, respectively, measured along the (010) direction as shown by the dashed green arrows in the insets. The black and red lines denote, respectively, the borders of the ST and BCT Brillouin zones. Blue curves in c and dashed brown curves in d are guides to the eye. In c the orange dashes mark the experimental location of the petals, whose intensity is too small to be apparent in this figure. ( e , f ) Raw energy distribution curves (EDCs) from ( c , d ) zooming into the region where the petals form. Spectra in blue correspond to k || =±| Q 1 |/2. ( g , h ) Same as c and d measured along (110) as shown by the dashed purple arrows in the insets. Dashed black lines are the Fermi momenta in the PM state. The blue curve in g is a fit serving as a guide to the eye [22] . ( i , j ) Raw EDCs from g and h . Spectra in blue show the Fermi momenta in the PM state. 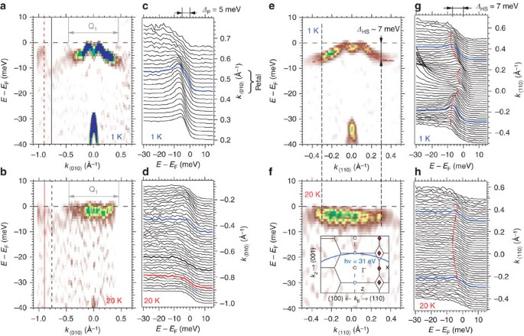Figure 3: Electronic gapping and reconstruction aroundZ. (a,b) ARPES dispersions (second derivative) along the (010) direction aroundZ, at respectively, 1 and 20 K. (c) Raw energy distribution curves (EDCs) from the spectra ina, zooming on the region where the Fermi petals form. The blue EDC corresponds tok||=±|Q1|/2. (d) Raw EDCs from the spectra inb, zooming on the region between the petals and the border of the BCT zone. The blue EDC corresponds tok||=±|Q1|/2, the bold black EDC is at the ST zone border and the red EDC is at the BCT zone border. It is noteworthy that the Fermi momentum here is sensibly smaller thank||=±|Q1|/2, showing that at 20 K the Fermi surface atZis different from the Fermi surface at Γ. (e,f) ARPES dispersions (second derivatives) at 1 and 20 K, respectively, measured along the (110) direction aroundZ. Dotted red lines are guides to the eye. (g,h) Raw EDCs corresponding to the spectra in (g,h). Spectra in blue correspond to the Fermi momenta of the PM state. Dotted red lines are guides to the eye. All data in this figure were measured athν=31 eV, corresponding to the spherical surface represented by the blue arc in the inset off. Full size image Figure 3 shows the associated changes in the electronic structure around Z , both along the (010) and (110) directions— Fig 3a–d and e–h , respectively. It is noteworthy that at 1 K, the spectra at Z , Fig. 3a,c,e,g , are essentially identical to the spectra at Γ, Fig. 2c,e,g,i . In both cases, one observes the central M-shaped band giving rise to the two inner Fermi squares, the small Fermi petals formed by the two-band anti-crossing at k ‹100› =±| Q 1 |/2, with an anti-crossing gap of 5 meV and the gap of 7 meV at hotspots of momenta k F ≈±0.3 Å −1 along (110). At 20 K, Fig. 3b,d,f,h , the states around Z disperse through E F , closing the previous gaps. Owing to the broad line shapes at this temperature, we cannot determine the precise shape of the Fermi sheet around Z in the PM state. Note however, from Fig. 3b,d , that the Fermi momenta around Z along (010) are now ~0.06 Å −1 smaller than | Q 1 |/2, their value around Γ along the same direction in the PM state. As we will discuss in detail later, these observations indicate that the electronic structures around Z and Γ become equivalent in the HO state. Figure 3: Electronic gapping and reconstruction around Z . ( a , b ) ARPES dispersions (second derivative) along the (010) direction around Z , at respectively, 1 and 20 K. ( c ) Raw energy distribution curves (EDCs) from the spectra in a , zooming on the region where the Fermi petals form. The blue EDC corresponds to k || =±| Q 1 |/2. ( d ) Raw EDCs from the spectra in b , zooming on the region between the petals and the border of the BCT zone. The blue EDC corresponds to k || =±| Q 1 |/2, the bold black EDC is at the ST zone border and the red EDC is at the BCT zone border. It is noteworthy that the Fermi momentum here is sensibly smaller than k || =±| Q 1 |/2, showing that at 20 K the Fermi surface at Z is different from the Fermi surface at Γ. ( e , f ) ARPES dispersions (second derivatives) at 1 and 20 K, respectively, measured along the (110) direction around Z . Dotted red lines are guides to the eye. ( g , h ) Raw EDCs corresponding to the spectra in ( g , h ). Spectra in blue correspond to the Fermi momenta of the PM state. Dotted red lines are guides to the eye. All data in this figure were measured at hν =31 eV, corresponding to the spherical surface represented by the blue arc in the inset of f . Full size image The spectral gaps at the hotspots and Fermi petals, Δ HS and Δ P , are further analysed and summarized in Fig. 4 . The raw energy distribution curves at the hotspots at 20 and 1 K are shown by the red and blue circles in Fig. 4a . The continuous lines under these data are fits using a Lorentzian spectral function (shadowed red and blue curves) plus a linear background, cut-off by a Fermi–Dirac distribution at the corresponding temperature, all convolved to a Gaussian of full-width at half maximum=5 meV, representing the experimental resolution broadening. This analysis shows that with respect to the Lorentzian at 20 K, the Lorentzian at 1 K sharpens and develops a gap Δ HS =6±1 meV. The leading-edge gap of ~2 meV results merely from resolution broadening. For comparison, the orange and green circles in Fig. 3a show the raw spectra along (110) at the outer square, at 20 and 1 K, respectively. At this k -point, the spectra sharpen but do not develop a gap in the HO state, as demonstrated by the leading edge of the raw data and the fits (orange and green continuous lines and shadowed Lorentzians). 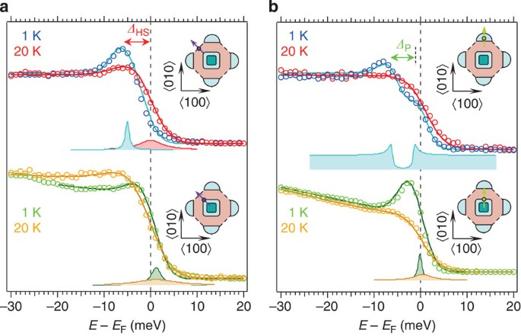Figure 4: Summary of energy gaps at the Fermi petals and hotspots. (a) Red and blue circles show the raw spectra at a hotspot (purple point in the schematic Fermi surface of the upper inset) in the PM and HO states, respectively. The continuous lines under the data are fits using a resolution-broadened Lorentzian spectral function (see text). The shadowed red and blue curves show the peaks resulting from the fits. The orange and green circles, lines and shadowed curves show the raw spectra, fits and Lorentzian peaks along (110) at the outer square (purple point in the lower inset) at 20 and 1 K, respectively. (b) Analogous toaat the Fermi petals (upper plots and green point in the schematic upper Fermi surface) and the outer square along (010) (lower plots and point in the schematic lower Fermi surface). The shadowed blue curve is a function of the form, (intrinsic broadening exaggerated in the plot), with singularities atE=Ec±ΔP/2, which, empirically, fits best the data in conjunction with the Fermi–Dirac distribution and the resolution broadening. The spectra were obtained by integrating the photoemission signal over 0.02 Å−1, which represents 1.3% of the ST Brillouin zone size. Figure 4: Summary of energy gaps at the Fermi petals and hotspots. ( a ) Red and blue circles show the raw spectra at a hotspot (purple point in the schematic Fermi surface of the upper inset) in the PM and HO states, respectively. The continuous lines under the data are fits using a resolution-broadened Lorentzian spectral function (see text). The shadowed red and blue curves show the peaks resulting from the fits. The orange and green circles, lines and shadowed curves show the raw spectra, fits and Lorentzian peaks along (110) at the outer square (purple point in the lower inset) at 20 and 1 K, respectively. ( b ) Analogous to a at the Fermi petals (upper plots and green point in the schematic upper Fermi surface) and the outer square along (010) (lower plots and point in the schematic lower Fermi surface). The shadowed blue curve is a function of the form , (intrinsic broadening exaggerated in the plot), with singularities at E = E c ± Δ P /2, which, empirically, fits best the data in conjunction with the Fermi–Dirac distribution and the resolution broadening. The spectra were obtained by integrating the photoemission signal over 0.02 Å −1 , which represents 1.3% of the ST Brillouin zone size. Full size image On the other hand, as shown in Fig. 4b for the data along (010), while the spectra at the outer square only sharpen in the HO state, the spectra at the petals’ centroid both sharpen and develop a double-peak structure. Empirically, we found that a function representing two Lorentzian-broadened, asymmetric singularities, separated by a gap Δ P , reproduces the 1 K data at the petals much better than any fit using a double Lorentzian (see Supplementary Fig. 2 and Supplementary Note 2 ). For both types of fits, the peak-to-peak gap is Δ P =5±1 meV. At 20 K, the double structure disappears and the local spectrum at the petals’ centroid is essentially described by a featureless Fermi–Dirac distribution. Symmetry change of the electronic structure The HO transition is also accompanied by conspicuous symmetry changes of the electronic structure. Note first, from Fig. 2a,b , that although at 1 K the spectral weights of the Fermi surfaces around Γ and Z are similar, at 20 K they are inequivalent, being more pronounced along (100) at Γ, and enhanced along (110) at Z . In fact, as noted earlier, in the HO state the heavy-band dispersions at Γ and Z are identical, but become dissimilar in the PM state. This suggests that below T HO , the electronic structure becomes consistent with a periodicity given by the commensurate vector Q 0 . It is noteworthy that these changes occur on heating the sample above T HO , and thus are not related to possible different photoemission selection rules at 50 and 31 eV, which are temperature-independent. Consider next the Brillouin-zone edge along (110). At hν =50 eV, this corresponds to a point, henceforth noted , located slightly below X , within 10% of the zone size along k z —see the inset of Fig. 2b . Fig. 5a,b show zooms around the left-most points of the Fermi surface maps in Fig. 2a,b . Although defining a precise shape of the Fermi surface around is difficult, as at this point the bands near E F are very heavy [22] , the data in Fig. 5a,b show a reconstruction of the spectral weight taking place across the transition, which we discuss below. 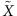Figure 5: Symmetry change from BCT to ST at thepoint. (a) Zoom around thepoint of the in-plane Fermi surface map at 20 K, measured athν=50 eV. The blue dashed ovals are guides to the eye. (b) Corresponding map at 1 K. The distribution of spectral weight aroundbecomes compatible with buckles closing around the borders of the ST zone. These result from the electronic ordering through a vectorQ0, folding the spectral weight of neighbouringpoints on top of each other (blue and green dashed ovals). Inaandb, grey dash-dotted lines show the BCT Brillouin zone atkz=Γ, red lines (full and dashed, respectively) show the actual edges aroundforhν=50 eV (see also the inset between panels) and black lines (dashed and full, respectively) the edges of the ST zone. Arrows labelled 1–4 show the direction of cuts across, presented incandd. (c) Momentum distribution curves at 20 K (red lines) and 1 K (blue lines) The zero in abscissas corresponds to thepoint. (d) Momentum distribution curves at 20 K (red lines) and 1 K (blue lines) along lines 3 and 4, parallel to ‹100› and ‹010›, respectively. The zero in abscissas corresponds to thepoint. Figure 5: Symmetry change from BCT to ST at the point. ( a ) Zoom around the point of the in-plane Fermi surface map at 20 K, measured at hν =50 eV. The blue dashed ovals are guides to the eye. ( b ) Corresponding map at 1 K. The distribution of spectral weight around becomes compatible with buckles closing around the borders of the ST zone. These result from the electronic ordering through a vector Q 0 , folding the spectral weight of neighbouring points on top of each other (blue and green dashed ovals). In a and b , grey dash-dotted lines show the BCT Brillouin zone at k z =Γ, red lines (full and dashed, respectively) show the actual edges around for hν =50 eV (see also the inset between panels) and black lines (dashed and full, respectively) the edges of the ST zone. Arrows labelled 1–4 show the direction of cuts across , presented in c and d . ( c ) Momentum distribution curves at 20 K (red lines) and 1 K (blue lines) The zero in abscissas corresponds to the point. ( d ) Momentum distribution curves at 20 K (red lines) and 1 K (blue lines) along lines 3 and 4, parallel to ‹100› and ‹010›, respectively. The zero in abscissas corresponds to the point. Full size image To try to rationalize the changes around , we represent by dashed ovals, in Fig. 5a , Fermi pockets compatible with the observed distribution of spectral weight at 20 K and matching the local two-fold symmetry of the body-centred tetragonal (BCT) zone. In the HO state, we expect the electronic structure to fold into a simple-tetragonal Brillouin zone, such that all the points become four-fold symmetric, and mutually perpendicular ovals on nearest-neighbour corners fold on each other. This results in an outer circle and an inner four-ring buckle, compatible with the Fermi-surface spectral weight observed at 1 K in Fig. 5b . It is noteworthy that a portion of the outer circle is also observed in the upper-left Fermi surface at 1 K in Fig. 2a . To check the above analysis, we plot in Fig. 5c,d the momentum distribution curves for the spectral weight at E F along lines 1 (parallel to Z − X − Z ), 2 (parallel to Γ− X −Γ or ‹110›), 3 (upper buckle) and 4 (left buckle) of Fig. 5a,b . It is noteworthy that for the cuts along lines 1 and 2, the spectral intensities are symmetric with respect to both at 20 K (red lines) and 1 K (blue lines), as these cuts correspond to high-symmetry directions in both the BCT and simple-tetragonal (ST) zones. A gap in spectral intensity at the is evident at 1 K, but not at 20 K. By contrast, along cuts 3 and 4, the spectral intensity is asymmetric with respect to at 20 K, corresponding to the distribution of spectral weight at E F observed in Fig. 5a , but it becomes symmetric with respect to at 1 K, compatible with an ST symmetry and the buckles observed in Fig. 5b . Note, from Fig. 5a,b , that the observed spectral intensity at 1 K is not symmetric with respect to the ST Brillouin zone for all cuts parallel to lines 3 and 4. In fact, as one can see from these figures, the spectral weight of the folded buckles at 1 K is largest where the original, unfolded features, were located at 20 K. This is qualitatively compatible with the coherence factors describing the momentum distribution of the spectral function in a standard band-folding or nesting scenario [26] , [27] . However, as it is presently unknown whether the HO state corresponds to a conventional density wave, and how the coherence factors should be calculated, a quantitative explanation of the observed distribution of spectral weight at E F lies beyond the scope of this work. In any case, from the data of Fig. 5 , it is clear that in the HO state the spectral weight is pushed to the other side of the ST zone edge, where it was not present in the PM state, strongly suggesting a symmetry change in the electronic structure from BCT to ST below T HO . It is noteworthy that this cannot be a temperature effect, as cooling down should have the opposite effect, namely, sharpening the spectral features and making the asymmetries more pronounced. The reconstruction of the 3D electronic structure from BCT to ST should also lead to a change of the Fermi-surface symmetry in the a − c plane—green plane in Fig. 1a . 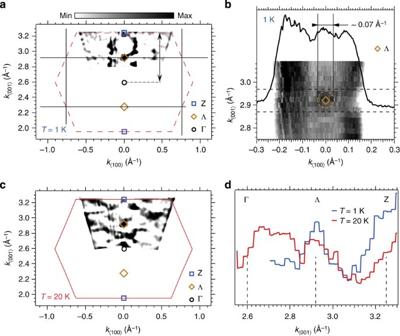Figure 6: Hidden-order changes in the electronic structure along (001). (a) Fermi surface map in the (100)−(001) plane at 1 K. The double arrow defines the ST periodicity alongc. Black lines define the ST Brillouin zone, while red dashed lines show the BCT zone. (b) Evidence of a new Fermi sheet around Λ: the ‘lentil’. The orange dashed oval is a guide to the eye. The black curve shows the intensity integrated between the two black dashed lines on the Fermi map. (c) Fermi surface map in the (100)−(001) plane at 20 K. The red lines show the BCT Brillouin zone. (d) Spectral weight atEFaroundk‹100›=0 alongk‹001›, both in the HO (blue) and PM (red) states. All data in this figure were obtained by varying the photon energy from 20 to 33 eV. The Fermi-surface maps inaandcare second derivatives, widely used in ARPES literature to enhance the signal-to-background ratio. These produce unphysical narrow strips of high intensity at the edges of the measured map, which were truncated inaandc. The corresponding complete raw data is shown in theSupplementary Fig. 3. The MDCs indwere integrated from the raw data associated toaandcover the intervalk‹100›=±0.05 Å−1. Figure 6 presents the measurements corresponding to this independent cross-check. As shown in Fig. 6a , in the HO state the two central Fermi sheets originating from the tips of the M-shaped heavy band present a dispersion along (001). Thus, although in the a − a plane these sheets have a square section, in the a − c plane they form concentric quasi-circles that cross almost tangentially at Λ, the midpoint between Γ and Z along (001). This dispersion along (001) demonstrates formally the bulk character of these two bands and, most important, shows that at 1 K the Fermi surface in the a − c plane is symmetric with respect to Λ. This suggests again that the 3D electronic structure shows a ST symmetry in the HO state, regardless of the underlying BCT crystal symmetry. Figure 6: Hidden-order changes in the electronic structure along (001). ( a ) Fermi surface map in the (100)−(001) plane at 1 K. The double arrow defines the ST periodicity along c . Black lines define the ST Brillouin zone, while red dashed lines show the BCT zone. ( b ) Evidence of a new Fermi sheet around Λ: the ‘lentil’. The orange dashed oval is a guide to the eye. The black curve shows the intensity integrated between the two black dashed lines on the Fermi map. ( c ) Fermi surface map in the (100)−(001) plane at 20 K. The red lines show the BCT Brillouin zone. ( d ) Spectral weight at E F around k ‹100› =0 along k ‹001› , both in the HO (blue) and PM (red) states. All data in this figure were obtained by varying the photon energy from 20 to 33 eV. The Fermi-surface maps in a and c are second derivatives, widely used in ARPES literature to enhance the signal-to-background ratio. These produce unphysical narrow strips of high intensity at the edges of the measured map, which were truncated in a and c . The corresponding complete raw data is shown in the Supplementary Fig. 3 . The MDCs in d were integrated from the raw data associated to a and c over the interval k ‹100› =±0.05 Å −1 . Full size image Incidentally, as the quasi-circles described above meet at Λ, they appear to hybridize, forming an inner small ‘Fermi lentil’ of diameter ~0.07±0.02 Å −1 , zoomed in Fig. 6b . On the other hand, the Fermi petals present a very weak intensity in these measurements along (001). Their exact dispersion and size in k z are difficult to infer from our data and remain open issues for future works. At 20 K, Fig. 6c , the a − c Fermi surface reconstructs and is not anymore symmetric with respect to Λ. The clearest feature at this temperature is a large rhombohedral Fermi surface, mostly located in the upper third of the BCT Brillouin zone, elongated along (100). Similar Fermi sheets dispersing quasi-linearly towards Γ and Z are also observed. From their momenta at these two points, those Fermi sheets would correspond to the large in-plane diamond-like Fermi surface observed in the PM state, described previously. Figure 6d shows the distribution of spectral weight at the Fermi level at k ‹100› =0 along k ‹001› , both at 1 and 20 K. From this figure, one also sees that the spectral weight is symmetric with respect to Λ in the HO state, but not in the PM state, further supporting the change of electronic symmetry from BCT at 20 K to ST at 1 K. Correspondence with thermo-transport data We now compare our data to transport and thermodynamic experiments to show how our measurements provide a unified microscopic picture of all the macroscopic changes induced by the HO transition. The extremal cross-sections, effective masses and electronic contribution to the specific heat γ e = C / T of several Fermi-surface sheets in the HO state have been previously determined by de-Haas–van Alphen and Shubnikov–de-Haas (SdH) measurements [7] , [15] . In Table 1 we compare our ARPES data to those transport results (details of the calculations in the Methods). We find an excellent correspondence between our data and the SdH measurements if we identify the outer central square with SdH’s α -sheet, the inner central square with the γ -sheet, the petals with the β -sheet and the lentil at Λ with the η -sheet. It is noteworthy that the SdH data as a function of field orientation of ref. 15 show that the cross-sectional area of the α -, γ - and η -sheets remains single-valued when sweeping the field from (001) to (100), compatible with central Fermi surfaces, while the β -sheet splits in two. By crystal symmetry, this sheet must then correspond to a Fermi surface with four non-central flattened pockets along the main axes of the Brillouin zone, exactly as the petals revealed by our experiments. Thus, our data in the HO state are fully compatible with SdH measurements, while providing a direct microscopic image of the 3D electronic structure of URu 2 Si 2 , including the PM state, not accessible through SdH. Table 1 SdH versus ARPES measurements. Full size table The transition from the large diamond-like Fermi surface around Γ to the four small petals occurs through the opening of a large gap of Δ HS ≈7 meV that suppresses ~70% of this Fermi sheet in the HO state ( Table 1 ). Together with the change in effective mass between the diamond and the petals, this implies a drastic reduction in the electronic contribution to the specific heat, as , where is the momentum-averaged effective mass of the Fermi sheet and S F its maximal cross-sectional area [15] . Hence, for the diamond-like Fermi surface alone, the change in electronic specific heat is γ e HO /γ e PM ≈0.4 ( Table 1 ). This agrees well with thermodynamic measurements, which show a dramatic entropy loss with a reduction in the Sommerfeld coefficient of γ e HO / γ e PM ≈(65 mJ × (mol × K 2 ) −1 /112 mJ × (mol × K 2 ) −1 )=0.58 induced by a gap opening of about 10 meV (ref. 3 ). Comparison between ARPES and band-structure calculations We finally compare, in Fig. 7a,b , the ARPES in-plane Fermi surfaces around Γ in the HO and PM states with the Fermi sheets in the large-moment antiferromagnetic (LMAF) and PM phases from the LDA calculations of ref. 12 . It is noteworthy that in those calculations the authors assume that the Brillouin zone folds from BCT to ST in the HO state, such that the Fermi surface in the HO state should be similar to the one computed for the LMAF phase. 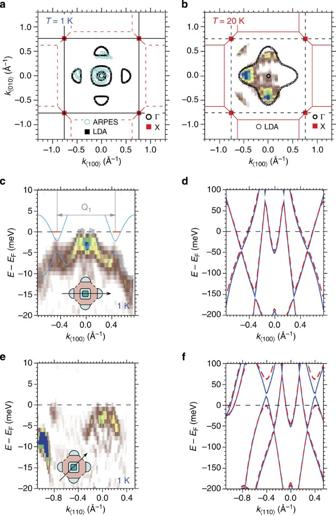Figure 7: Comparison between ARPES and LDA in thea−aplane around Γ. (a) Fermi momenta from our ARPES data in the HO state (open blue circles) and LDA calculations of the Fermi surface in the LMAF state (black squares, from ref.12). The electronic structure in the LMAF and HO states are assumed to be similar by the authors of such calculations. (b) Experimental (colour plot, second derivative of ARPES data) and LDA (circles, ref.12) Fermi surfaces around Γ in the PM state. (c,d) Experimental and LDA dispersions in the HO state along (100), as shown in the inset ofc. The data incare the same as inFig. 2c. The blue and red lines in the LDA calculations correspond to the PM and LMAF states, respectively. (e,f) Similar tocanddalong the (110) direction. Figure 7: Comparison between ARPES and LDA in the a − a plane around Γ. ( a ) Fermi momenta from our ARPES data in the HO state (open blue circles) and LDA calculations of the Fermi surface in the LMAF state (black squares, from ref. 12 ). The electronic structure in the LMAF and HO states are assumed to be similar by the authors of such calculations. ( b ) Experimental (colour plot, second derivative of ARPES data) and LDA (circles, ref. 12 ) Fermi surfaces around Γ in the PM state. ( c , d ) Experimental and LDA dispersions in the HO state along (100), as shown in the inset of c . The data in c are the same as in Fig. 2c . The blue and red lines in the LDA calculations correspond to the PM and LMAF states, respectively. ( e , f ) Similar to c and d along the (110) direction. Full size image As can be concluded from these figures, there is a good agreement between the experimental and local-density approximation (LDA) Fermi surfaces. In the HO state, the inner and outer central squares and the four non-central Fermi petals observed by ARPES correspond well with the LDA Fermi sheets in the LMAF state. In addition, when going to the PM state, the calculations show a gap closing around (110), as observed in the ARPES measurements at the hotspot (main text), producing in both cases similar diamond-like Fermi sheets—albeit the calculated Fermi sheet appears slightly larger than the experimental one. Thus, these agreements between the ARPES data and LDA calculations are another strong indication that, below T HO , the electronic structure follows an ST symmetry. On the other hand, as shown in Fig. 7c,e , the experimental electronic structure near E F in the HO phase shows bands dispersing over only a few meV and energy gaps over this same energy scale. By contrast, the purely itinerant LDA calculations, Fig. 7d,f , give dispersions and energy gaps over energy scales at least one order of magnitude larger [12] . In fact, a detailed comparison between the experimental band dispersion at 1 K along (100), Fig. 7c , and the corresponding LDA dispersion, Fig. 7d , shows a reasonable agreement between the shapes of the bands near E F , but with an experimental effective mass ten times larger, given by the factor in energy scales needed to overlap the theoretical and experimental dispersions. This large mass renormalization, resulting from the heavy f -states that govern the low-energy band masses of URu 2 Si 2 , is taken into account by other theories or calculations based on a dual local-itinerant approach [13] , [24] , [20] . An additional notable difference between the experimental and LDA dispersions along (100) is that at the petals, the data show the anti-crossing-like 5 meV gap, while in the calculations the band-crossing yielding the petals is not avoided, neither in the PM nor in the HO states. The comparison between the experimental and LDA band dispersions at 1 K along the (110) direction, Fig. 7d, e , shows more marked differences. For instance, although the LDA calculations predict a band anti-crossing at around k ‹110› =0.4 Å −1 , with a gap of ~60 meV separating an upper unoccupied electron pocket and a lower occupied hole pocket with its maximum right at E F , the data show a gap Δ HS ≈7 meV with respect to E F at this position, and no sign of a hole pocket, or a band anti-crossing, in the vicinity of this k -point. Note again a factor of ~10 between the energy scales of the measured and calculated dispersions. Other ARPES experiments with lower energy resolution performed only at T < T HO reported a decrease of spectral weight at E F around Γ along the (110) direction, and an increase along (100), with respect to states at binding energies larger than 100 meV (ref. 28 ). Here, our results unambiguously show that the regions of depleted spectral weight are in fact strongly gapped at E F in the HO state with respect to the PM state, due to the Fermi-surface reconstruction from the large diamond to the small petals, and from a BCT to a ST symmetry. Other recent high-resolution ARPES experiments also reported a gap opening of 7 meV along the (110) direction, and suggested a change to an ST symmetry in the HO state [29] , but the survey of the electronic structure was limited to the spectra at the Γ and Z points. It is noteworthy that the extensive gapping of the large diamond Fermi surface, shown by our data, implies the suppression, in the HO state, of a large volume of Fermi momenta available for scattering. This naturally explains the abrupt increase in the electron lifetime below T HO observed by previous thermal transport and ARPES experiments [14] , [30] , and studied in detail in another recent ARPES work [31] . Our results show that the most prominent macroscopic and microscopic signatures of the HO transition are all the result of a massive reconstruction of a heavy-fermion Fermi surface, that we directly image here for the first time. Furthermore, the fact that the periodicity of the electronic structure in the HO state is well described by Q 0 indicates that this vector, and not Q 1 , is directly related to the HO parameter—thus, strongly limiting the number of viable theories for the HO transition. The energy gaps at Q 1 and along the hot arcs would then be an outcome of the above electronic reconstruction. An analogous situation is encountered in electron-doped cuprates, in which band-folding by a commensurate antiferromagnetic wave vector creates gaps at incommensurate wave vectors [27] . In addition, our determination of the multi-band Fermi-surface topology in the HO state should provide crucial input for the experimental and theoretical understanding of the superconducting order parameter in URu 2 Si 2 (ref. 32 ), to which the HO is a precursor. Finally, the similarities and differences between the data, measured in the HO state, and the calculations, formally in the LMAF state, might have a significance in the understanding of the HO transition, and should be further studied experimentally and theoretically. More generally, our results are the first direct determination of a momentum-dependent Fermi-surface gapping in a heavy-fermion system, opening bright perspectives for future studies of exotic classic and quantum phase transitions in these materials. Sample preparation and measurements The high-quality URu 2 Si 2 single crystals were grown in a tri-arc furnace equipped with a Czochralski puller, and subsequently annealed at 900 °C under ultrahigh vacuum for 10 days. The high-resolution ARPES experiments were performed with a Scienta R4000 detector at the UE112-PGM-1b (‘1 3 ’) beamline of the Helmholtz Zentrum Berlin—BESSY-II using horizontally polarized light from hν =16 eV (total instrument resolution ~4 meV) to hν =50 eV (resolution ~7 meV). The samples were cleaved in situ along the (001) plane at 1 K. The pressure was below 5 × 10 −11 Torr throughout the measurements. All Fermi-surface maps in this work were obtained by integrating the ARPES data over E F ±1 meV. The experimental Fermi momenta were determined from fits to momentum distribution curves at E F . The results have been reproduced in five different cleaves. Lattice parameters and reciprocal-lattice units URu 2 Si 2 has a BCT crystal structure, of base side a =4.12 Å and height c =9.68 Å. Thus, a *≡2 π / a =1.52 Å −1 , and the length of the vector Q 1 is | Q 1 |=(1±0.4) × a *, giving 2.135 Å −1 or 0.915 Å −1 . 3D k -space mapping Within the free-electron final state model, ARPES measurements at constant photon energy give the electronic structure at the surface of a spherical cap of radius . Here, m e is the free electron mass, Φ is the work function and V 0 =13 eV is the ‘inner potential’ of URu 2 Si 2 (refs 8 , 14 , 22 ). Measurements around normal emission provide the electronic structure in a plane nearly parallel to the a − a plane, as those presented in Figs 1 and 2 . Likewise, measurements as a function of photon energy provide the electronic structure in the a − c plane, presented in Fig. 6 . Second derivative rendering For second-derivative rendering, the raw photoemission intensity maps were convolved with a two-dimensional Gaussian of widths σ E =3 meV and σ k =0.02 Å −1 for T =1 K, and σ E =4 meV and σ k =0.03 Å −1 for T =20 K. The corresponding figures in this work show the negative values of the second derivative along the energy axis, which represent peak maxima in the original energy distribution curves. Characteristics of Fermi sheets from ARPES data For a Fermi-surface sheet of area S F , we define the average Fermi momentum such that: as done in SdH works [15] . For electron-like Fermi sheets (diamond, petals and inner square), we note E 0 the bottom of the band, directly determined from the ARPES data, and define the average effective mass such that: For instance, for the inner square ( γ -sheet), we have and E 0 ≈4 meV, which gives . We obtain independent consistent values of the effective masses of the electron-like Fermi sheets through parabolic fits to their dispersions along the (100) and (110) directions. To estimate the mass of the hole-like outer square, we fitted the whole M-shaped band around Γ or Z using a three-band model with interband hybridization, introduced in our previous work [22] , and extracted the band mass around E F from the curvature of the fitted dispersion at E F . As a byproduct, we obtained again a value of the effective mass of the inner electron-like square that agrees with the parabolic estimate for this band. In addition, a simple hole-like parabolic fit to the dispersion of the outer square in the vicinity of E F gives an effective mass that is compatible with the result of the full fit to the M-shaped structure. Finally, from the average Fermi momenta and effective masses, we calculated, following ref. 15 , the Sommerfeld coefficient associated to each Fermi sheet as: where k B is Boltzmann constant and V =49 cm 3 mol −1 is the molar volume of URu 2 Si 2 . It is noteworthy that, for the effective mass and Sommerfeld coefficient of the diamond-like Fermi surface in the PM state, we considered only the electron-like dispersion around Γ and neglected the crossing with the other band at k ‹100› =±| Q 1 |/2. There is indeed a difficulty in how to estimate, from the present ARPES data, the Sommerfeld coefficient of the diamond-like Fermi sheet in the PM state. The exact calculation depends on the details of the two bands crossing near E F , such as the energy at which they cross with respect to E F or whether they rather maintain the anti-crossing gap at 20 K, and on the momentum-dependence of this crossing around the Fermi surface. For instance, from our data, the crossing of the bands along (110) is not evident, suggesting that the effect of such crossing on the effective masses along the whole diamond Fermi sheet would be negligible. However, these details remain challenging for future experiments. In any case, the Sommerfeld coefficient of the diamond-like Fermi surface alone cannot exceed the total Sommerfeld coefficient in the PM state observed by thermodynamic measurements, which is ~120 mJ mol −1 K −2 (ref. 3 ), or twice our estimate of the Sommerfeld constant for this Fermi sheet. Thus, our calculation of γ e HO / γ e PM ≈40% is, at worst, underestimating by a factor of 2 the loss in specific heat for the diamond Fermi surface. This will be attenuated by the fact that a large part of this ‘missing’ factor 2 in the PM state should come from the Fermi sheets around Z and X , whose Sommerfeld coefficients at 20 K are difficult to evaluate from our present data. How to cite this article: Bareille, C. et al . Momentum-resolved hidden-order gap reveals symmetry breaking and origin of entropy loss in URu 2 Si 2 . Nat. Commun. 5:4326 doi: 10.1038/ncomms5326 (2014).